Long non-coding RNA Gm15441 attenuates hepatic inflammasome activation in response to PPARA agonism and fasting Exploring the molecular mechanisms that prevent inflammation during caloric restriction may yield promising therapeutic targets. During fasting, activation of the nuclear receptor peroxisome proliferator-activated receptor α (PPARα) promotes the utilization of lipids as an energy source. Herein, we show that ligand activation of PPARα directly upregulates the long non-coding RNA gene Gm15441 through PPARα binding sites within its promoter. Gm15441 expression suppresses its antisense transcript, encoding thioredoxin interacting protein (TXNIP). This, in turn, decreases TXNIP-stimulated NLR family pyrin domain containing 3 (NLRP3) inflammasome activation, caspase-1 (CASP1) cleavage, and proinflammatory interleukin 1β (IL1B) maturation. Gm15441 -null mice were developed and shown to be more susceptible to NLRP3 inflammasome activation and to exhibit elevated CASP1 and IL1B cleavage in response to PPARα agonism and fasting. These findings provide evidence for a mechanism by which PPARα attenuates hepatic inflammasome activation in response to metabolic stress through induction of lncRNA Gm15441 . There is growing support for a strong link between metabolism and inflammation [1] , [2] . Various fasting regimes are known to provide many health benefits, including anti-inflammatory effects [3] . Peroxisome proliferator-activated receptor α (PPARα) is a ligand-activated nuclear receptor and transcription factor that is a key regulator of fatty acid oxidation and the fasting response. PPARα facilitates metabolic remodeling that promotes lipid oxidation, and its dysregulation contributes to metabolic disorders and liver disease [4] . Prolonged activation by the PPARα-specific ligand WY-14643 has many phenotypic characteristics that parallel the fasting response [5] , [6] , [7] , [8] . Metabolic changes that promote fat oxidation can lead to metabolic stress through increased lipid peroxidation and reactive oxygen species generation, both of which are known pro-inflammatory signals [9] , [10] . Interestingly in the context of elevated fatty acid oxidation, several synthetic PPARα agonists, including WY-14643, act as potent anti-inflammatory agents [11] . However, the regulatory mechanisms underlying how PPARα prevents inflammation are not well understood. Long non-coding RNAs (lncRNAs) act as regulators of gene expression and play important regulatory roles in many metabolic processes. For example, lncRNA Blnc1 works in concert with another important hepatic nuclear receptor, liver X receptor (LXR), to activate the lipogenic gene program [12] . Downregulation of lncRNA lncOb reduces leptin, leading to a leptin responsive form of obesity [13] . Other studies found that lncRNAs are regulated during adipocyte differentiation [14] , [15] , are expressed in the liver in a sex-dependent manner when regulated by growth hormone [16] , [17] , and can be strongly induced by xenobiotic exposure [18] . A compartment-specific transcriptional profiling approach revealed that lncRNA PAXIP1-AS1 regulates pulmonary arterial hypertension by modulating smooth muscle cell function [19] . Further, lncRNA HOTAIR influences glucose metabolism by upregulation of GLUT1 in hepatocellular carcinoma cells [20] . It is, therefore, reasonable to consider that lncRNAs may play important roles in the metabolic remodeling and anti-inflammatory actions that occur after PPARα activation. Thioredoxin interacting protein (TXNIP) acts as a critical relay linking oxidative and endoplasmic reticulum (ER) stress to inflammation through NLR family pyrin domain containing 3 (NLRP3) inflammasome activation [21] . NLRP3 inflammasome activation is a two-step process. The first step involves inflammasome assembly and is referred to as “priming”. At this stage the inflammasome is waiting to be “activated” by diverse stimuli including ionic flux, lysosomal damage, mitochondrial dysfunction, and, notably, oxidative stress [22] , [23] , [24] . These signals then trigger inflammasome activation resulting in caspase cleavage and cleavage of target proteins such as pro-inflammatory cytokines. TXNIP is bound intracellularly to thioredoxin and plays a role in oxidative stress-induced NLRP3 inflammasome activation [25] . As oxidative stress increases, thioredoxin is released from TXNIP freeing it to associate with the NLRP3 inflammasome. Several studies have shown that elevated TXNIP expression impacts NLRP3 inflammasome activation and cleavage of caspase-1 (CASP1) to the mature, proteolytically active p20 form [21] , [26] , [27] . Mature CASP1 (p20) then cleaves interleukin 1β (IL1B) precursor to the active pro-inflammatory cytokine. Studies have also indicated that NLRP3 inflammasome activity is attenuated by mono- and polyunsaturated fatty acids, which are endogenous PPARα agonists [28] , [29] . RNA-seq data presented here revealed that lncRNA Gm15441 , an antisense lncRNA of Txnip , is robustly increased by PPARα activation. The primary Gm15441 transcript is spliced, generating a mature RNA composed of four exons. Two of the four exons directly overlap with exonic regions of the Txnip gene. Antisense transcripts often interact the corresponding sense transcripts encoded from the opposing gene, thereby interfering with post-transcriptional control by promoting transcript degradation or disrupting translation [30] . The Gm15441 transcript was identified through several independent transcriptome profiling studies providing support that this may be a functionally important lncRNA [31] , [32] , [33] . Using siRNA, one study found that Gm15441 knockdown by siRNA impacted hepatocyte fatty acid oxidation in vitro, however, the mechanism was not determined [31] . In the current study, the mechanisms by which the PPARα target lncRNA Gm15441 prevents inflammation during periods of metabolic stress were investigated. ChIP-seq datasets were analyzed for PPARα binding sites within the Gm15441 promoter, and Gm15441 regulatory elements were confirmed using reporter gene assays and PPARα ChIP studies. Gm15441 transgene expression downregulated Txnip , demonstrating lncRNA-mediated gene suppression in vitro. CRIPSR/Cas9-mediated gene editing was employed to develop a Gm15441 knockout ( Gm15441 LSL ) mouse model. Basal TXNIP levels in Gm15441 LSL mice were significantly elevated over wild-type mice, supporting the role of Gm15441 as a negative regulator of Txnip expression in vivo. Gm15441 LSL mice were treated with a PPARα agonist or fasted to assess how loss of Gm15441 impacts hepatic inflammasome activation in response to both pharmacological and physiologically-induced metabolic stress. TXNIP protein, active cleaved CASP1 levels, and IL1B cleavage were elevated in Gm15441 LSL mice, and were further increased by PPARα activation, indicating that this lncRNA plays a major role in attenuating inflammasome activation. Thus, hepatic PPARα directly regulates the lncRNA Gm15441 , which in turn suppresses Txnip expression, attenuating NLRP3 inflammasome activation during periods of metabolic stress. Together, these findings support a regulatory mechanism whereby fatty acids mobilized from adipose tissue during fasting activate PPARα, which in turn suppresses the NLRP3 inflammasome by strong induction of the TXNIP-suppressing antisense lncRNA gene Gm15441 . Thus, these studies reveal a regulatory mechanism supporting the beneficial effects of fasting, namely, reduced inflammation. LncRNA regulation by PPARα is highly tissue-specific To assess the regulation of lncRNAs by PPARα, RNA-seq was performed using total liver RNA isolated from Ppara +/+ and Ppara −/− mice, both with and without dietary exposure to the PPARα agonist WY-14643. A lncRNA discovery pipeline was implemented that identified 15,558 liver-expressed lncRNA genes. Of these, 13,343 were intergenic, 1966 were antisense to known coding genes, and 249 were intragenic lncRNAs. Forty-four percent of the 15,558 liver-expressed lncRNAs are considered novel [17] . Differential gene expression analysis revealed that a total of 1735 RefSeq genes and 442 liver-expressed lncRNA genes responded to treatment with WY-14643 at an expression fold-change > 2 at FDR < 0.05, with 968 RefSeq genes and 245 lncRNA genes upregulated, and 767 RefSeq genes and 197 lncRNA genes downregulated following WY-14643 treatment (Supplementary Data 1 and 2 ). Only 17 RefSeq genes (1.0%) and six lncRNAs (1.3%) responded to WY-14643 in the same manner in Ppara -null mice. Thus, ~99% of these transcriptomic responses are PPARα-dependent (Fig. 1a ). Fig. 1: LncRNA identified as PPARα targets are expressed in several oxidative tissues but exhibit liver-specific transcriptional response to WY-14643. a Venn diagrams of RefSeq transcripts and lncRNA transcripts that were differentially regulated by WY-14643 (fold change > 2 at FDR < 0.05) in wild-type and in Ppara −/− mouse liver, as determined by RNA-seq. 123 of the RefSeq genes are non-coding, indicated by their NR accession numbers. Six RefSeq genes and six lncRNA genes show opposite responses to WY-14643 treatment and are excluded from the gene counts shown. b Relative basal lncRNA expression in select tissues. c LncRNA expression in tissues from Ppara +/+ and Ppara −/− mice treated with WY-14643 for 48 h. At least five mice were analyzed for each genotype and treatment group. Each bar represents the mean ± SD for n = 5 tissue samples. Adjusted p values, provided in the panels, as determined by ANOVA with Tukey’s multiple comparison correction, one-sided for comparisons to Ppara +/+ mice or as shown (dashed horizontal lines). ND not detected. Full size image Comparison of the PPARα-responsive lncRNAs to lncRNAs responsive to agonist ligands of two other nuclear receptors in mouse liver, namely CAR and PXR [18] , identified eight lncRNAs that are induced by all three nuclear receptors and 11 lncRNAs repressed by all three receptors. Forty-five other lncRNAs were induced, or were repressed, in common by PPARα and CAR, and 30 other lncRNAs were either induced or repressed in common by PPARα and PXR (Supplementary Data 3 ). Overall, 94 (21%) of the 442 PPARα-responsive liver-expressed lncRNAs showed common responses to CAR and/or PXR activation. Furthermore, 59 other PPARα-responsive lncRNAs showed opposite patterns of response to PPARα as compared to CAR or PXR (Supplementary Data 3 ). These findings are consistent with the partial functional overlap between these three xenobiotic nuclear receptors and their gene targets [34] , [35] , [36] . 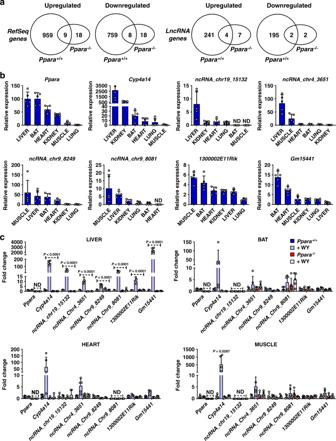Fig. 1: LncRNA identified as PPARα targets are expressed in several oxidative tissues but exhibit liver-specific transcriptional response to WY-14643. aVenn diagrams of RefSeq transcripts and lncRNA transcripts that were differentially regulated by WY-14643 (fold change > 2 at FDR < 0.05) in wild-type and inPpara−/−mouse liver, as determined by RNA-seq. 123 of the RefSeq genes are non-coding, indicated by their NR accession numbers. Six RefSeq genes and six lncRNA genes show opposite responses to WY-14643 treatment and are excluded from the gene counts shown.bRelative basal lncRNA expression in select tissues.cLncRNA expression in tissues fromPpara+/+andPpara−/−mice treated with WY-14643 for 48 h. At least five mice were analyzed for each genotype and treatment group. Each bar represents the mean ± SD forn= 5 tissue samples. Adjustedpvalues, provided in the panels, as determined by ANOVA with Tukey’s multiple comparison correction, one-sided for comparisons toPpara+/+mice or as shown (dashed horizontal lines). ND not detected. Pathway analysis revealed that the WY-14643 upregulated genes are most highly enriched for the following biological processes: lipid metabolism, peroxisome, DNA replication, DNA repair, cell cycle, and fatty acid oxidation (Supplementary Table 1 ). 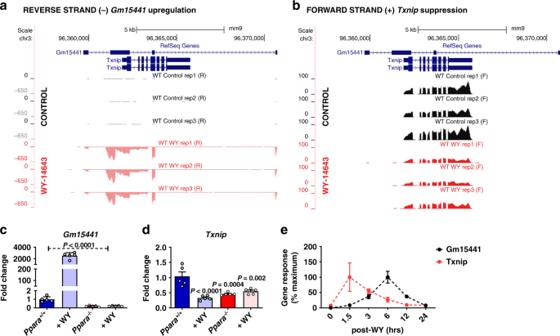Fig. 2:Txnipand lncRNAGm15441are inversely regulated following PPARα activation. Wild-type (Ppara+/+) mice were treated with WY-14643 and stranded RNA-seq was performed on total liver mRNA.aExpression of the antisense lncRNAGm15441is strongly upregulated.bExpression of the protein-codingTxnipmRNA is downregulated. Shown are the changes in expression ofGm15441(c), andTxnip(d), mRNAs inPpara+/+andPpara−/−mice treated with WY-14643, or vehicle control, for 48 h, determined by qRT-PCR.eTime course for changes in expression ofGm15441andTxnipmRNA over a 24 h period following treatment with WY-14643 by gavage, determined by qRT-PCR. The maximum response ofTxnipmRNA was seen at 1.5 h and forGm15441was seen at 6 h. Each data point represents the mean ± SD forn= 5 liver samples. Adjustedpvalues, provided in the panels, as determined by ANOVA with Tukey’s multiple comparison correction, two-sided for comparisons toPpara+/+mice or as shown (dashed horizontal line). The downregulated genes are most highly enriched for: secreted factors, monooxygenase, immunity, serine protease inhibitor, metabolism of xenobiotics, and response to virus (Supplementary Table 2 ). PPARα-dependent lncRNAs identified by RNA-seq were selected and mRNA levels monitored over a 24-h period after WY-14643 treatment, revealing that lncRNA expression profiles paralleled those of known protein-coding PPARα target genes (Supplementary Fig. 1a–d ). As lncRNA expression is often highly tissue specific [16] , [37] , [38] , the relative basal levels were measured for PPARα-responsive lncRNAs expressed in oxidative tissues that utilize fatty acids as an energy source and express PPARα at the highest levels. Ppara mRNA and its classic target gene Cyp4a14 served as controls. Basal levels of Cyp4a14 mRNA and intergenic lncRNAs ncRNA_chr19_15132 and ncRNA_chr4_3651 were highest in liver, while ncRNA_chr9_8249, ncRNA_chr9_8081 , and 1300002E11Rik were most highly expressed in muscle. One of the PPARα-dependent lncRNAs, Gm15441 , was also most highly expressed in brown adipose tissue (BAT) (Fig. 1b ). To assess the impact of PPARα activation on lncRNA expression and tissue specificity, Ppara wild-type mice ( Ppara +/+ ) and Ppara -null mice ( Ppara −/− ) were treated with WY-14643 for 48 h, and four tissues (liver, BAT, heart, muscle) then harvested for analysis. Cyp4a14 mRNA was markedly induced by WY-14643 in all four tissues and in a Ppara -dependent manner, as expected (Fig. 1c ). All six lncRNAs were induced in liver, including Gm15441 , which exhibited >2000-fold increase in wild-type livers, more than 10-fold higher than the other lncRNAs. In contrast to the induction of Cyp4a14 mRNA, lncRNA induction by WY-14643 was liver-specific, with no significant induction of the five other lncRNAs seen in BAT, heart, or muscle (Fig. 1c ). Further, none of these lncRNAs was induced in Ppara −/− mice in any tissue examined. Thus, PPARα-mediated induction of these lncRNAs is highly liver-specific, with Gm15441 showing the most robust induction response. LncRNA Gm15441 is antisense to Txnip and exhibits inverse regulation in response to PPARα activation LncRNA Gm15441 overlaps the coding region of Txnip , which is located on the opposing strand and responds to WY-14643 treatment, albeit with different kinetics than Gm15441 (see below). Bioinformatic analysis confirmed that Gm15441 lacks coding potential and was categorized as a non-coding transcript (Supplementary Fig 2a, b ). Analysis of the mapped sequence reads obtained by stranded RNA-sequencing revealed a pronounced increase in expression of Gm15441 (Fig. 2a ), whereas, the Txnip transcript on the opposite strand was suppressed by WY-14643 at the 48-hour time point analyzed (Fig. 2b ). Rapid amplification of cDNA ends (RACE) results showed that the primary hepatic Gm15441 transcript exon-exon boundaries matched the current annotation of Gm15441 (NR_040409.1) (Supplementary Fig. 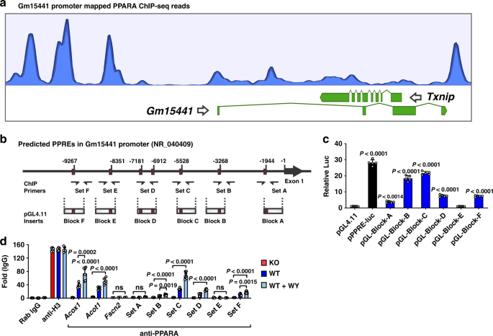Fig. 3: LncRNAGm15441is a direct PPARα target gene. aPPARα ChIP-seq read peaks from agonist (GW7647)-treated mouse liver.bSchematic representation of seven PPRE sequences found within theGm15441promoter (−10 kb). ChIP primer binding sites and reporter gene construct inserts are shown.cLuciferase-based reporter assays identified several functional PPREs within theGm15441promoter, based onn= 3 replicates.dPPARα ChIP assays assessed PPRE binding in liver samples fromPpara+/+andPpara−/−mice treated with WY-14643. Experiments were performed with at least four different livers. Rabbit IgG and antibody to histone H3 were used as negative and positive controls, respectively. Each data point represents the mean ± SD forn= 5 liver samples. Adjustedpvalues, provided in the panels, as determined by ANOVA with Tukey’s multiple comparison correction, one-sided for comparisons to pGL4.11 empty vector (c) or as indicated (d). ns not significant. 3a and Supplementary Table 3 ). Gene and isoform structures analysis for mouse liver Gm15441 by de novo transcriptome assembly using CuffMerge identified three isoforms of Gm15441 (Supplementary Fig. 3b ). The second isoform (TCONS_00330193) is identical to the RefSeq gene isoform, the first isoform is a splice variant, and the third isoform has an alternative third exon and is missing exon 4 (Supplementary Fig. 3b ). All three isoforms share the precise 5′ end, two full length isoforms share a common 3′ end (Supplementary Fig. 3c, d ). qRT-PCR analysis confirmed the very large, highly significant increase in Gm15441 expression and its complete inhibition in Ppara −/− liver (Fig. 2c ). Further, Txnip RNA levels were significantly suppressed by WY-14643 in wild-type mice (Fig. 2d ). Additionally, Txnip expression was attenuated in untreated Ppara −/− compared to Ppara +/+ mouse liver, indicating a role for PPARα in maintaining basal expression of Txnip (Fig. 2d ). Given that Txnip expression can be upregulated in human neuroblastoma cells by the PPARα activator fenofibrate, which suppresses proliferation and migration [39] , the effects of a single dose of WY-14643 on Gm15441 and Txnip mRNA were examined over a 24 h period. Txnip mRNA was induced rapidly, with maximum expression seen at 1.5 h, followed by a marked decrease coincident with the increased expression of Gm15441 (Fig. 2e ). Inverse regulation of Txnip mRNA and Gm15441 RNA were also observed in response to fasting (Supplementary Fig. 4 ). These time courses are markedly different from those of 14 other WY-14643-inducible protein-coding and lncRNA genes examined, where peak induction occurred 6–12 h after WY-14643 treatment (Supplementary Fig. 1 ), as was also found for Gm15441 . The unusual kinetics seen with Txnip —early induction followed by repression coinciding with the activation of Gm15441 —indicate that Txnip is a PPARα target gene whose expression in liver is inversely regulated with that of Gm15441 after PPARα activation. Reporter assays confirmed that the Txnip promoter region has functional PPARα regulatory elements that overlap the sites of PPARα binding detected by ChIP-seq (Supplementary Fig. 5a, b ). Fig. 2: Txnip and lncRNA Gm15441 are inversely regulated following PPARα activation. Wild-type ( Ppara +/+ ) mice were treated with WY-14643 and stranded RNA-seq was performed on total liver mRNA. a Expression of the antisense lncRNA Gm15441 is strongly upregulated. b Expression of the protein-coding Txnip mRNA is downregulated. Shown are the changes in expression of Gm15441 ( c ), and Txnip ( d ), mRNAs in Ppara +/+ and Ppara −/− mice treated with WY-14643, or vehicle control, for 48 h, determined by qRT-PCR. e Time course for changes in expression of Gm15441 and Txnip mRNA over a 24 h period following treatment with WY-14643 by gavage, determined by qRT-PCR. The maximum response of Txnip mRNA was seen at 1.5 h and for Gm15441 was seen at 6 h. Each data point represents the mean ± SD for n = 5 liver samples. Adjusted p values, provided in the panels, as determined by ANOVA with Tukey’s multiple comparison correction, two-sided for comparisons to Ppara +/+ mice or as shown (dashed horizontal line). Full size image PPARα directly regulates lncRNA Gm15441 by binding to its promotor To identify PPARα binding sites at the Gm15441 / Txnip locus, PPARα ChIP-seq datasets (GSE61817) from PPARα agonist-treated mice [40] were analyzed (Fig. 3a ). Three major ChIP-seq peaks, indicating PPARα binding, were seen upstream of Gm15441 , and one major peak was seen in the promoter region of Txnip . Examination of genomic sequences upstream of Gm15441 using Genomatix MatInspector (Genomatix, Munich, Germany) identified seven peroxisome proliferator response elements (PPREs) within six genomic regions, designated A to F, within 10 kilobase (kb) upstream of the Gm15441 transcriptional start site (TSS) (Fig. 3b ). These six Gm15441 upstream sequences were synthesized and cloned into the pGL4.11 reporter, and luciferase assays were performed to assay the functionality of PPARα binding to the Gm15441 promoter. A PPRE-luciferase construct containing an Acox1 PPRE repeat was used as a positive control, and an empty pGL4.11 plasmid was used as a negative control. Luciferase activity was significantly elevated in primary mouse hepatocytes transfected with five of the six pGL4.11 constructs, consistent with direct regulation by PPARα at multiple loci (Fig. 3c ). PPARα binding was also assessed by ChIP assays using a polyclonal PPARα antibody and chromatin isolated from livers of wild-type and Ppara −/− mice fed either control diet or a diet containing WY-14643. Enrichment of PPARα binding to PPREs of known PPARα target genes, namely Acot1 and Acox1 , was determined by comparing binding to liver chromatin from wild-type mice fed control diet vs. WY-14643-containing diet (Fig. 3d ). Ppara −/− livers were used as a negative control to identify non-specific binding. Fscn2 primers were used as a non-target gene promoter and negative control. Enrichment of PPARα binding was found using primer sets covering Gm15441 regions B, C, D, and F, while no binding was seen with Gm15441 region E (Fig. 3d ), which was transcriptionally inactive (Fig. 3c ). Enrichment was strongest with region C, in agreement with the luciferase reporter gene data. Enrichment at sites C and D was significantly increased by WY-14643 treatment, indicating increased PPARα recruitment at these sites. No PPARα binding was seen with chromatin from Ppara −/− mice on the control diet. Together, these data indicate that PPARα regulates Gm15441 transcription by direct binding of PPARα to multiple PPRE sites within 10 kb of the Gm15441 TSS. Fig. 3: LncRNA Gm15441 is a direct PPARα target gene. a PPARα ChIP-seq read peaks from agonist (GW7647)-treated mouse liver. b Schematic representation of seven PPRE sequences found within the Gm15441 promoter (−10 kb). ChIP primer binding sites and reporter gene construct inserts are shown. c Luciferase-based reporter assays identified several functional PPREs within the Gm15441 promoter, based on n = 3 replicates. d PPARα ChIP assays assessed PPRE binding in liver samples from Ppara +/+ and Ppara −/− mice treated with WY-14643. Experiments were performed with at least four different livers. Rabbit IgG and antibody to histone H3 were used as negative and positive controls, respectively. Each data point represents the mean ± SD for n = 5 liver samples. Adjusted p values, provided in the panels, as determined by ANOVA with Tukey’s multiple comparison correction, one-sided for comparisons to pGL4.11 empty vector ( c ) or as indicated ( d ). ns not significant. Full size image Generation of a strand-specific Gm15441 knockout mouse A gene targeting strategy was developed to generate a Gm15441 knockout mouse without impacting Txnip expression on the opposing strand. To accomplish this goal, CRISPR/Cas9 was used to insert a Lox-STOP-Lox (LSL) cassette downstream of Gm15441 exon 1 (Fig. 4a, b ). The LSL cassette prevents transcription of Gm15441 in a Gm15441 -floxed mouse but has no effect on transcription of Txnip , which is inserted >2 kb downstream of the last exon of Txnip . Crossing with a transgenic Cre mouse deletes the LSL cassette and restores Gm15441 expression (Fig. 4c ). All mouse lines were on a pure C57BL/6J background. The genotyping scheme generates an approximately 1200 bp band in Gm15441 wild-type mice ( Gm15441 +/+ ) and a 1700 bp band in Gm15441 LSL mice (Fig. 4d ). Basal expression of Gm15441 was neglectable in livers of Gm15441 LSL when compared to Gm15441 +/+ mice (Fig. 4e ). Expression in heterozygous Gm15441 HET mice was comparable to Gm15441 LSL . To verify the subcellular localization and loss of expression of Gm15441 , fluorescence in situ hybridization (FISH) staining was performed on livers from Gm15441 +/+ and Gm15441 LSL mice fed control diet or treated with WY-14643. DAPI staining was used as a counter stain to detect nuclei in liver sections. A pronounced increase in Gm15441 fluorescence was detected in the cytoplasm and nuclei of hepatocytes in livers from WY-14643-treated Gm15441 +/+ mice. The Gm15441 RNA signal was absent in livers from vehicle-treated Gm15441 +/+ and Gm15441 LSL mice, and in livers from WY-14643-treated Gm15441 LSL mice (Fig. 4f ). Gm15441 transcript copy number was determined to be around 100 RNA molecules per hepatocyte (Supplementary Fig. 6a, b ). These data validate Gm15441 LSL mice as an effective knockout mouse model and reveal that hepatic Gm15441 expression is both nuclear and cytosolic evoking several possible mechanisms by which it regulates Txnip . Fig. 4: Generation of the Gm15441 -null mouse line. Targeting strategy for generating a strand-specific Gm15441 -null mouse line. a Exon structure of the targeted Gm15441 - Txnip locus. b CRISPR/Cas9-mediated insertion of Lox-STOP-Lox (LSL) cassette selectively ablates Gm15441 expression. c Cre-mediated removal of STOP cassette rescues Gm15441 expression. d Gm15441 knockout mouse genotyping. e Analysis of Gm15441 RNA by qRT-PCR from livers of Gm15441 +/+ , Gm15441 +/− , and Gm15441 LSL mice. Each data point represents the mean ± SD for n = 5 liver samples. Adjusted p values, provided in the panels, as determined by ANOVA with Tukey’s multiple comparison correction, one-sided for comparisons to Gm15441 +/+ mice. f Representative fluorescence in situ hybridization staining of Gm15441 RNA in livers of Gm15441 +/+ and Gm15441 LSL mice treated with WY-14643 for 48 h ( n = 5, 3 images/mouse). Scale bars represents 20 nm (×200). Full size image Loss of Gm15441 potentiates inflammasome activation by WY-14643-induced metabolic stimulation PPARα plays a role in attenuating inflammation in many tissues and disease models [41] , [42] . In the liver, PPARα ameliorates inflammation by reducing ER stress in hepatocytes [43] . TXNIP is known to facilitate ER stress-induced NLRP3 inflammasome activation [27] , [44] . By regulating TXNIP levels, Gm15441 could serve as a link between PPARα and the NLRP3 inflammasome. To ascertain whether lncRNA Gm15441 attenuates inflammasome activation by regulating TXNIP levels, mice were treated with WY-14643 for 48 h, and weight loss, liver index (mg liver/g total body mass), ALT, AST, and serum glucose levels were measured. There was no discernable difference in weight loss between Gm15441 +/+ and Gm15441 LSL mice on a WY-14643 diet (Fig. 5a ). Serum ALT and AST levels were unchanged by genotype or following WY-14643 treatment. Serum glucose levels were significantly decreased by WY-14643 in both Gm15441 +/+ and Gm15441 LSL mice, but the decrease was significantly greater in Gm15441 LSL mice (Fig. 5a ). However, insulin and glucose tolerance tests, performed on Gm15441 LSL mice, indicate that these animals are insulin sensitive (Supplementary Fig. 7a–d ). Furthermore, pronounced hepatomegaly was induced by WY-14643 treatment in both Gm15441 +/+ and Gm15441 LSL mice, as indicated by the significant increase in liver size (Fig. 5a , liver index), and by the pronounced swelling of hepatocytes seen by H&E staining (Fig. 5b ). Expression of the PPARα target genes acyl-CoA dehydrogenase medium chain ( Acadm ) and Cyp4a14 was significantly increased by WY-14643 in both Gm15441 +/+ and Gm15441 LSL mice. Gm15441 was strongly upregulated in livers of wild-type mice but was not detected in Gm15441 LSL mice. Txnip mRNA was significantly decreased by WY-14643 in livers of wild-type animals, consistent with Fig. 2 , but was significantly induced in Gm15441 LSL livers (Fig. 5c ). There was also a small but significant increase in Il1b mRNA expression in wild-type mice treated with WY-14643 (Fig. 5d ). Basal levels of the inflammasome-related proteins TXNIP, cleaved CASP1 (p20), and cleaved IL1B were elevated in livers of Gm15441 LSL mice compared to wild-type mice, and further increased following WY-14643 treatment (Fig. 5e, f ). Overall, levels of all three proteins were much higher in livers of WY-14643-treated Gm15441 LSL mice than wild-type mice (Fig. 5e ). To test whether TXNIP is responsible for the phenotype observed in Gm15441 LSL mice, an adenovirus associated virus (AAV) expressing short hairpin (sh) Txnip (AAV-shRNA- Txnip ) vector was generated. The AAV-shRNA- Txnip virus was injected into the tail vein of Gm15441 +/+ and Gm15441 LSL mice, and following a recovery period, the mice were placed on a control diet or WY-14643-containing diet for 24 h. WY-14643-induced liver indices and histological changes were not affected by Txnip knockdown (Supplementary Fig. 8a, b, g ). Txnip mRNA and protein expression were suppressed by Txnip knockdown, or by WY-14643 treatment, in Gm15441 +/+ mice (Supplementary Fig. 8a, c, d ); they were also suppressed by Txnip knockdown in WY-14643-treated Gm15441 LSL mice (Supplementary Fig. 8b, e, f ). Cleaved CASP1 and IL1B protein were significantly suppressed by Txnip knockdown in WY-14643-treated Gm15441 +/+ mice, but not in WY-14643-treated Gm15441 LSL mice (Supplementary Fig. 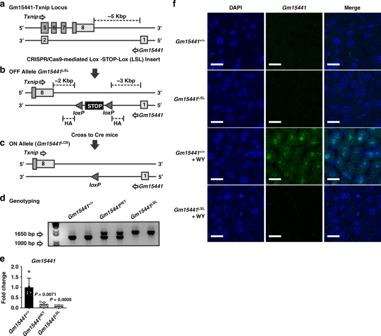Fig. 4: Generation of theGm15441-null mouse line. Targeting strategy for generating a strand-specificGm15441-null mouse line.aExon structure of the targetedGm15441-Txniplocus.bCRISPR/Cas9-mediated insertion of Lox-STOP-Lox (LSL) cassette selectively ablatesGm15441expression.cCre-mediated removal of STOP cassette rescuesGm15441expression.dGm15441knockout mouse genotyping.eAnalysis ofGm15441RNA by qRT-PCR from livers ofGm15441+/+,Gm15441+/−, andGm15441LSLmice. Each data point represents the mean ± SD forn= 5 liver samples. Adjustedpvalues, provided in the panels, as determined by ANOVA with Tukey’s multiple comparison correction, one-sided for comparisons toGm15441+/+mice.fRepresentative fluorescence in situ hybridization staining of Gm15441 RNA in livers ofGm15441+/+andGm15441LSLmice treated with WY-14643 for 48 h (n= 5, 3 images/mouse). Scale bars represents 20 nm (×200). 8c–f and Supplementary Table 4 ). These data support the view that Gm15441 plays an important role in WY-14643 induced metabolic stress in the liver. Thus, the ablation of Gm15441 increases the expression of TXNIP and maturation of two other proteins associated with NLRP3 inflammasome activation, namely, cleaved CASP1 and IL1B. Fig. 5: Loss of Gm15441 potentiates inflammasome activation by WY-14643. a Physiological endpoints from Gm15441 +/+ and Gm15441 LSL mice treated with WY-14643 for 48 h. Weight loss and liver indices (mg liver/g body mass; a measure of hepatomegaly), as well as serum ALT, AST, and glucose levels, in response to WY-14643 treatment. b Representative H&E staining from liver of Gm15441 +/+ and Gm15441 LSL mice treated with WY-14643 for 48 h ( n = 5, 3 images/mouse). Scale bars represent 100 nm (×400). c qRT-PCR analysis of Acadm , Cyp4a14 , Txnip , and Gm15441 expression in livers of mice treated with WY-14643 for 48 h. d qRT-PCR analysis of Il1b and Casp1 mRNA in livers of mice treated with WY-14643. e Western blot analysis of TXNIP, ACTB, CASP1 (cleaved), and IL1B (cleaved) protein in livers from mice treated with WY-14643 for 48 h. f Densitometric analysis of TXNIP, CASP1 (cleaved), and IL1B (cleaved) protein levels ( n = 3). Each data bar represents mean ± SD for n = 5 liver samples; red bars, WY-14643 treatment. Adjusted p values, provided in the panels, as determined by ANOVA with Tukey’s multiple comparison correction, two-sided for comparisons between WY-14643 and control livers of the same genotype, or as shown (dashed horizontal lines). Full size image Loss of Gm15441 potentiates inflammasome activation during physiological response to acute fasting During fasting, hepatic PPARα facilitates the metabolic remodeling that promotes use of lipids as an alternate energy source [4] . Fasting is also associated with many anti-inflammatory effects [3] . To determine whether Gm15441 regulates inflammasome activation during physiological fasting, Gm15441 +/+ and Gm15441 LSL mice were fasted for 24 h. Serum ALT and AST were not changed between Gm15441 +/+ and Gm15441 LSL mice, both with and without WY-14643 treatment (Fig. 6a ). Fasting decreased serum glucose levels in both Gm15441 +/+ and Gm15441 LSL mice, but the decrease was greater in Gm15441 LSL mice (Fig. 6a ). Expression of Acadm , Cyp4a14 , and Txnip mRNAs was significantly increased by fasting in both Gm15441 +/+ and Gm15441 LSL mice (Supplementary Fig. 9a ). Gm15441 was significantly induced by fasting, although to a much lower degree than with WY-14643 treatment (Supplementary Fig. 9a ). Expression of Txnip mRNA was increased to the same level in livers of fasted Gm15441 LSL mice as in fasted Gm15441 +/+ mice (Supplementary Fig. 9a ). Fasting also increased TXNIP, cleaved CASP1 (p20), and cleaved IL1B protein levels in Gm15441 LSL mice, in contrast to either a modest increase (TXNIP) or no increase (CASP1, IL1B) in Gm15441 +/+ mice (Supplementary Fig. 9b, c ). Fasting markedly promotes lipid accumulation in mouse liver [4] . Lipid droplet accumulation was also observed and more widespread in fasting Gm15441 LSL mice than fasting Gm15441 +/+ mice (Supplementary Fig. 9d ). Oil Red O staining was performed to validate lipid accumulation in response to fasting in Gm15441 LSL mice. A greater amount of lipid accumulation was observed in fasting Gm15441 LSL liver than in fasting Gm15441 +/+ mouse liver (Fig. 6b ). Expression of lipid metabolism-related genes was not significantly impacted in Gm15441 LSL mice under fasting conditions (Supplementary Fig. 10 ). Serum non-esterified fatty acids (NEFA), serum and liver triglyceride (TG) levels, and liver (but not serum) total cholesterol (CHOL) levels, were significantly elevated in fasting Gm15441 LSL mouse livers compared to fasting Gm15441 +/+ mouse livers (Fig. 6c ). 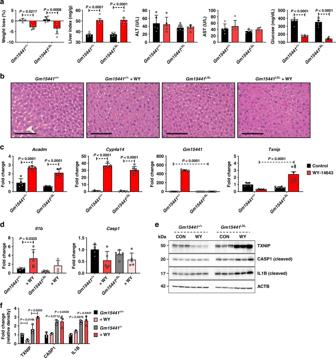Fig. 5: Loss ofGm15441potentiates inflammasome activation by WY-14643. aPhysiological endpoints fromGm15441+/+andGm15441LSLmice treated with WY-14643 for 48 h. Weight loss and liver indices (mg liver/g body mass; a measure of hepatomegaly), as well as serum ALT, AST, and glucose levels, in response to WY-14643 treatment.bRepresentative H&E staining from liver ofGm15441+/+andGm15441LSLmice treated with WY-14643 for 48 h (n= 5, 3 images/mouse). Scale bars represent 100 nm (×400).cqRT-PCR analysis ofAcadm,Cyp4a14,Txnip, andGm15441expression in livers of mice treated with WY-14643 for 48 h.dqRT-PCR analysis ofIl1bandCasp1mRNA in livers of mice treated with WY-14643.eWestern blot analysis of TXNIP, ACTB, CASP1 (cleaved), and IL1B (cleaved) protein in livers from mice treated with WY-14643 for 48 h.fDensitometric analysis of TXNIP, CASP1 (cleaved), and IL1B (cleaved) protein levels (n= 3). Each data bar represents mean ± SD forn= 5 liver samples; red bars, WY-14643 treatment. Adjustedpvalues, provided in the panels, as determined by ANOVA with Tukey’s multiple comparison correction, two-sided for comparisons between WY-14643 and control livers of the same genotype, or as shown (dashed horizontal lines). These findings were supported by RNA-sequencing analysis, which revealed that liver damage and lipid accumulation-related genes were impacted by Gm15441 deficiency, albeit in a complex manner (Supplementary Table 5 ). To check whether Gm15441 influences lipid mobilization or uptake, total lipase activity was measured in liver, skeletal muscle, and inguinal white adipose tissue (IWAT) from fed and fasted mice (Supplementary Fig. 11a–c ). Total lipase activity was elevated in the livers of fasted Gm15441 LSL mice (Supplementary Fig. 11a ). Total lipase activity in skeletal muscle was decreased by fasting in Gm15441 +/+ mice and fed or fasted Gm15441 LSL mice when compared to fed wild-type mice (Supplementary Fig. 11b ). However, the difference between fasted Gm15441 +/+ and Gm15441 LSL mice was not significant (Supplementary Fig. 11b ). Total lipid activity in IWAT was not significantly different between genotype with or without fasting (Supplementary Fig. 11c ). Furthermore, analysis of the impact of fasting on mRNAs for lipocalin 2 ( Lcn2 ), orosomucoid 2 ( Orm2 ), serum amyloid A1 ( Saa1 ), and serum amyloid A2 ( Saa2 ) – biomarker genes for liver damage, inflammation, and/or fatty accumulation – showed these genes were significantly elevated with fasting in Gm15441 LSL compared to Gm15441 +/+ mouse livers (Fig. 6d ). ELISA results indicated serum SAA1 levels were also significantly increased by fasting in Gm15441 LSL mice (Supplementary Fig. 12 ). Fasting induced lower but still significant increases in several of these mRNAs in Gm15441 +/+ livers, which could reflect the fasting-induced increase in Txnip expression (Supplementary Fig. 9a–d ). Thus, Gm15441 negatively regulates the NLRP3 inflammasome pathway and lipid accumulation, potentially by preventing Txnip expression, in response to fasting. Fig. 6: Loss of Gm15441 potentiates inflammasome activation during physiological response to acute fasting. a Physiological endpoints from Gm15441 +/+ and Gm15441 LSL mice after 24 h fasting. Weight loss and liver indices (mg liver/g body mass; a measure of hepatomegaly), as well as blood ALT, AST, and glucose levels, in response to fasting. b Representative ORO staining of liver tissues after a 24 h fed or fast in Gm15441 +/+ and Gm15441 LSL mice ( n = 5, 3 images/mouse). Scale bars represents 100 nm (×200). c Non-esterified fatty acid (NEFA) from serum, triglycerides (TG) and cholesterol (CHOL) levels from serum and liver tissues after a 24 h fast. d Analysis of Apoa4 , Bhmt , Lcn2 , Orm2 , Saa1 , and Saa2 mRNAs in livers of Gm15441 +/+ and Gm15441 LSL mice after 24 h fasting. Each data bar represents the mean ± SD for n = 5 liver samples; green bars, 24 h fasting. Adjusted p values, provided in the panels, as determined by ANOVA with Tukey’s multiple comparison correction, two-sided for comparisons between fast-stimulated and unstimulated livers of the same genotype, or as shown (dashed horizontal lines). Full size image Translational regulation of TXNIP by Gm15441 is partially dependent on 5′UTR sequences Translational regulation of TXNIP can occur via internal ribosome entry site (IRES) sequences found in the 5′UTR [45] . IRES sequences are commonly associated with cell survival- and stress response-related genes and utilized when cap-dependent translation is inhibited during nutrient deprivation [46] . The 5′UTR of Txnip contains binding sites for IRES trans-acting factors (ITAFs), which regulate IRES-mediated translation [45] . As Gm15441 transcription generates an RNA antisense to the 5′UTR of Txnip , Gm15441 RNA may block ITAF protein binding to the Txnip 5′UTR and thereby inhibit Txnip translation. To investigate this regulatory mechanism, the translational inhibitory potential of the Txnip 5′UTR was examined when linked to the coding sequence for GFP (Fig. 7a ). The GFP and the 5′UTR-GFP expression vectors were each transfected into Hepa-1 cells together with a Gm15441 expression vector or an empty expression plasmid. After 48 h, strong Gm15441 expression was achieved, but there were no effects on the RNA levels of GFP or UTR-GFP (Fig. 7b ). In contrast, GFP protein translated from the Txnip 5′UTR-GFP template was significantly reduced in cells co-transfected with Gm15441 expression plasmid (Fig. 7c ). This 5′UTR-dependent decrease in GFP protein was most striking when examined by fluorescent microscopy (Fig. 7d, e ). These findings suggest that Gm15441 regulates TXNIP translation through IRES sites found within its 5′UTR. In vitro transcription-translation assays performed using reticulocyte lysates provided additional evidence that Gm15441 directly suppresses TXNIP protein levels, whereby increasing Gm15441 expression levels caused a corresponding decrease in TXNIP protein expression (Supplementary Fig. 13a, b ). To examine whether lncRNA Gm15441 impacts expression of genes that flank Gm15441 on mouse chromosome 3, namely, Hfe2 (Hjv) , Pol3gl , and Ankrd34a , Hepa-1 and NIH3T3 mouse embryonic fibroblast cells were transfected with Gm15441 expression vector, or empty plasmid. The Gm15441 transgene was expressed and significantly downregulated Txnip without impacting the expression of Hfe2 , Pol3gl , or Ankrd34a (Fig. 7f ). Furthermore, TXNIP protein expression was suppressed by Gm15441 expression in vitro (Supplementary Fig. 14a, b ). Together, these data support a regulatory mechanism whereby PPARα induces Gm15441 , which in turn attenuates inflammation through TXNIP and the NLRP3 inflammasome pathway (Fig. 7g ). Fig. 7: Gm15441 regulates TXNIP translation in part through IRES sequences found within the 5′UTR of TXNIP. a Schematic representation of GFP construct inserts with or without the TXNIP 5′UTR sequence. b Analysis of Gm15441 RNA and Gfp mRNA in Hepa-1 cells. c Western blot analysis of GFP protein and relative density of GFP signal from Hepa-1 cells (right). d Fluorescence of GFP in Hepa-1 cells transfected with GFP with empty or Gm15441 plasmid DNA for 48 h ( n = 3). Scale bars represent 20 nm (100x). e Fluorescence of GFP in Hepa-1 cells transfected with 5′ UTR sequence containing GFP with empty or Gm15441 plasmid DNA for 48 h ( n = 3). Scale bars represent 20 nm (100x). f Analysis of Hfe2 , Pol3gl , and Ankrd34a mRNAs from Hepa-1 and NIHT3T cells transfected with empty plasmid or Gm15441 expression vector for 24 h. Each data point represents mean ± SD for n = 3 replicates. Adjusted p values, provided in the panels, as determined by ANOVA with Tukey’s multiple comparison correction, one-sided for comparisons in the absence of Gm15441 ( b , c ) or to empty vector ( f ). g Model for role of Gm15441 in suppressing TXNIP-mediated inflammasome activation. Full size image The physiological alterations that accompany fasting impart several health benefits, including anti-inflammatory effects [47] . PPARα activation during fasting is a key regulatory event of lipid and glucose metabolism. A growing body of evidence indicates that PPARα activation also potently suppresses inflammation in several disease models and tissues [48] . However, the mechanism by which PPARα modulates metabolic stress-induced inflammation is not known. The direct regulation of protein-coding genes by PPARα is well characterized, but it was not known whether lncRNAs – which may influence gene expression through a variety of mechanisms [49] —also serve as direct targets contributing to physiological changes induced by PPARα activation. The present study identified several hundred PPARα-responsive liver-expressed lncRNA genes including several antisense lncRNAs, which often contribute to the regulation of genes on the opposing strand [50] , [51] . Further, a PPARα-dependent regulatory axis involving one such antisense lncRNA, Gm15441 , was characterized. Gm15441 was shown to be transcribed in a liver-specific, PPARα-dependent manner to yield an antisense lncRNA that protects against metabolic stress by suppressing expression of the opposing sense transcript, TXNIP, and thereby suppresses TXNIP-mediated NLRP3 inflammasome activation. RNA-seq analysis of livers from wild-type and Ppara −/− mice treated with the PPARα-specific agonist WY-14643 identified more than 400 liver-expressed lncRNA transcripts that were significantly upregulated or downregulated 48 h after WY-14643 treatment. Only six of these lncRNAs were similarly responsive to WY-14643 in Ppara −/− mice, thus establishing the striking PPARα dependence of these non-coding RNA transcriptomic responses. PPARα-dependent, liver-specific expression was verified for six non-coding RNAs, and detailed functional studies were carried out on one such gene, Gm15441 , which showed an unusually strong induction in WY-14643-treated liver. Importantly, the genomic orientation of Gm15441 is antisense to that of Txnip . The Txnip gene encodes a ubiquitously-expressed protein that facilitates cellular responses to oxidative stress and inflammation [52] . TXNIP was originally identified as a negative regulator of thioredoxin [53] , and subsequent studies found that TXNIP contributes to a wide array of processes in several tissues. TXNIP is key regulator of NLRP3 inflammasome activation, which plays an important role in liver fibrosis and hepatocellular carcinoma [54] , and its activation is associated with the NLRP3 inflammasome pathway in human diseases [55] . TXNIP has also emerged as an important glucose sensor that regulates glucose uptake in response to insulin [56] and plays an important role in metabolic stress [57] , [58] . An earlier study found that Ppara mRNA and PPARα target gene mRNAs were elevated in Txnip -null mice, and that Txnip expression attenuated PPRE-luciferase activity when co-transfected with PPARα/RXR and treated with WY-14643 [59] , suggesting a Txnip-Ppara feedback regulatory loop that may also involve Gm15441 . LncRNAs regulate diverse cellular processes, including metabolism-related genes expressed on the opposing strand [60] . The present results showed that Gm15441 negatively regulates Txnip expression during metabolic stress. LncRNA Gm15441 is antisense to Txnip , whose mRNA is decreased in liver coincident with the robust increase in Gm15441 expression beginning 3 h after activation of PPARα by WY-14643. The underlying PPARα regulatory interactions controlling activation of the Gm15441 promoter were investigated, and several PPARα binding sites identified within 10 kb of the Gm15441 TSS were confirmed by ChIP assays and shown to be functional in reporter gene assays. Thus, the TXNIP antisense lncRNA Gm15441 is a direct target of PPARα in WY-14643-stimulated mouse liver. Pharmacological activation of PPARα deregulates NLRP3 inflammasome activity in a mouse model of diabetes [61] and prolonged hepatic NLRP3 inflammasome activation leads to hepatocyte death, inflammation, and fibrosis [62] , [63] . Mice treated solely with the PPARα agonist WY-14643 exhibit pronounced liver hepatomegaly, hepatocyte hypertrophy, and lipid accumulation. These changes are coupled to an increase in oxidative stress [64] . Oxidative stress is known to stimulate NLRP3 inflammasome activation and IL1B maturation [22] , [23] , [24] , [65] , [66] . Interestingly, differential gene expression and pathway analysis of RNA-sequencing data in wild-type mice treated solely with WY-14643 revealed activation of some acute inflammatory response pathways. Thus, the TXNIP-mediated NLRP3 inflammasome pathway was examined. Txnip mRNA was significantly decreased by PPARα activation in livers of wild-type and Gm15441 +/+ mice, while TXNIP protein was elevated in livers of Gm15441 LSL mice. Furthermore, TXNIP-mediated NLRP3 inflammasome activation resulted in cleavage of CASP1 to its mature, proteolytically active p20 form. Mature CASP1 subsequently cleaves target proteins, including the pro-inflammatory cytokine IL1B to its corresponding mature, active form. Mature, cleaved CASP1 (p20) and IL1B protein were elevated in Gm15441 LSL mice, indicating an increase in inflammasome activation. Thus, PPARα activation of lncRNA Gm15441 suppresses the TXNIP-mediated NLRP3 inflammasome pathway in response to metabolic stress. PPARα plays an important regulatory role in the fasted mouse liver model [4] . Hepatic expression of PPARα target genes Acadm and Cyp4a14 was significantly increased by fasting, as was the expression of Txnip mRNA, in livers of Gm15441 LSL mice as well as Gm15441 +/+ mice compared with fed mice. However, TXNIP protein was more highly increased in fasting Gm15441 LSL mice compared to fasting Gm15441 +/+ mice. Fasting Txnip mRNA levels are closely associated with lipid and glucose regulation [67] . In addition, TXNIP-mediated NLRP3 inflammasome pathway target protein cleavage (i.e., CASP1 and IL1B) was significantly elevated in livers of fasting Gm15441 LSL mice compared to Gm15441 +/+ mice. These results support the proposal that physiological upregulation of lncRNA Gm15441 in response to fasting prevents metabolic stress by suppressing the TXNIP-mediated NLRP3 inflammasome response. PPARα, a key regulator of global lipid homeostasis, modulates fasting-induced lipid accumulation and hepatosteatosis in mice [4] . Lipid droplets appeared in livers of fasted Gm15441 +/+ mice but were more widely distributed in livers of fasting Gm15441 LSL mice. Histological lipid staining revealed considerably larger amounts of lipid accumulation in livers of fasted Gm15441 LSL mice than in wild-type mouse livers. Moreover, serum and liver TG levels and liver CHOL levels were also significantly elevated by fasting in Gm15441 LSL mice. To determine whether Gm15441 influences lipid mobilization or uptake, total lipase activity was measured in liver, skeletal muscle, and inguinal white adipose tissue (IWAT) from fed and fasted Gm15441 +/+ and Gm15441 LSL mice. Total lipase activity in liver was elevated in fasted Gm15441 LSL mice after 24 h while fasting didn’t affect lipase levels in wild-type mice. Elevated hepatic lipase activity in fasted Gm15441 LSL mice is suggestive of an increase in lipid uptake. As lipids and TGs in the liver accumulate, spillover into circulation would be expected and may explain the observed increase. Lipase activity in the skeletal muscle of fed Gm15441 LSL mice was significantly lower than wild-type suggesting Gm15441 may influence lipid uptake into this tissue. Interestingly, our data shows that basal Gm15441 expression levels are considerably higher in skeletal muscle than liver suggesting that this lncRNA may have yet-to-be determined functions within other non-hepatic tissues. RNA-seq analysis revealed that liver damage, inflammation, and fatty accumulation biomarkers such as Lcn2 , Orm2 , Saa1 , and Saa2 mRNAs showed significantly higher expression under fasting-induced metabolic stress in Gm15441 LSL compared to wild-type. Hepatic Lcn2 and Orm2 mRNAs are both upregulated in the liver in response to IL1B [68] , [69] . SAA1 and SAA2 are major acute phase proteins which are activated in response to inflammation [70] . Activation is dependent on proteolytic cleavage by matrix metallopeptidases (MMPs), namely MMP9 [71] . Hepatic MMP9 expression is responsive to IL1B activation [72] . Therefore, the increase in SAA1 and SAA2 further substantiates elevated NLRP3-induced inflammation in our model. Like SAA1 and SAA2, OSM2 is an acute phase protein associated with inflammation that is primarily produced in the liver [73] . Although the exact function of this protein has not been discovered, elevation of its expression is linked to several inflammatory diseases, suggesting that it is an important marker of inflammation [73] , [74] , [75] , [76] . Lipocalin-2 (LCN2) is also specifically associated with NLRP3 inflammasome activation [77] . The increase in mature, cleaved IL1B in Gm15441 LSL mice may at least partially explain the increased hepatic expression of Lcn2, Orm2, Saa1 , and Saa2 mRNAs in fasted Gm15441 LSL mice. Thus, these genes are all associated with inflammation/oxidative stress, consistent with the PPARα-dependent attenuation by Gm15441 of TXNIP-associated hepatic inflammation in response to metabolic stress. IRES is an RNA element that allows for translation initiation of certain mRNAs, including TXNIP, when cap-dependent translation is inhibited under stress conditions [45] . ITAFs such as polypyrimidine tract binding protein were shown to regulate TXNIP expression during nutrition starvation by binding to IRES sequences within the Txnip 5′UTR [45] . By binding to these IRES sequences, ITAF proteins regulate translation initiation and TXNIP protein expression. As lncRNA Gm15441 is antisense to TXNIP and its exon 3 almost entirely overlaps the Txnip 5′UTR, Gm15441 may block IRES sequences needed for translation of TXNIP. The ability of Gm15441 to modulate TXNIP protein levels via Txnip 5′UTR IRES sequences was demonstrated in vitro by co-transfection of a GFP reporter with a Gm15441 expression vector. A decrease in GFP expression was dependent on both Gm15441 and the Txnip 5′UTR, indicating that Gm15441 in part regulates TXNIP through its 5′UTR, presumably by masking functional IRES sites. In vitro transcription-translation assays provided additional evidence that Gm15441 directly suppresses TXNIP protein levels. Incrementally increasing Gm15441 expression caused a corresponding decrease in TXNIP protein suggesting that translation was repressed. Together, these data support a mechanism whereby Gm15441 translationally regulates TXNIP protein levels through IRES sites found within the TXNIP 5′UTR. The strand-specific Gm15441 knockout mouse developed in this study enabled us to assess the function of this lncRNA without impacting regulation of its antisense protein-coding partner, Txnip . In contrast, previous knockout mouse models developed to evaluate TXNIP function disrupt both Txnip and Gm15441 , and therefore abolish the unique regulatory loop that exists between these two genes. Txnip -null mice show a higher incidence of hepatocellular carcinoma, with approximately 40% of male mice developing hepatic tumors [78] . However, the Txnip -null mice lack exons 1–4, and thus Gm15441 is also ablated [79] . TXNIP expression in vitro inhibited hepatocellular carcinoma cell proliferation and induced apoptosis [80] . Thus, prolonged Gm15441 -mediated suppression of TXNIP may also contribute to PPARα agonist induced hepatocellular carcinoma [81] . In summary, the present study focused on the role of lncRNAs as potential metabolic regulators. Pharmacological activation of PPARα promoted induction of large numbers of hepatic lncRNAs, a subset of which are also targeted by the nuclear receptors CAR and PXR. Gm15441 was identified as a liver-specific, PPARα-dependent lncRNA positioned antisense to the pro-inflammatory gene Txnip . Gm15441 expression was shown to suppress TXNIP protein by a mechanism involving the blocking of IRES sites within its 5′UTR. By suppressing TXNIP translation, Gm15441 inhibited TXNIP-mediated activation of the NLRP3 inflammasome as well as subsequent CASP1 cleavage and IL1B maturation. Taken together, these results demonstrate that lncRNA Gm15441 can directly prevent metabolic stress-induced inflammation and represents a therapeutic target for the treatment of inflammatory disorders. Mouse models Male 8- to 12-week-old mice were used for all studies and all mouse strains were on the C57BL/6J background and maintained on a grain-based control diet (NIH-31). Mice were housed in light (12 h light: 12 h darkness cycle) and temperature-controlled rooms (humidity 40–60%) and were provided with water and pelleted chow ad libitum . For pharmacological studies, the mice were provided a grain-based control diet or matched diet containing 0.1% WY-14643 for 24 or 48 h. For monitoring the time dependence of gene responses, WY-14643 was dissolved in 1% carboxymethyl cellulose (CMC) solution and orally administered by gavage (50 mg/kg in 200 μl). At the end of the treatment period, the mice were killed by CO 2 asphyxiation and tissues harvested. For physiological studies, food was removed for 24 h starting shortly after the onset of the light cycle and endpoints collected at the same time the following day. Animals were then killed, and tissue samples harvested for further analysis. Blood was collected by venipuncture of the caudal vena cava. All animal experiments were performed in accordance with the Association for Assessment and Accreditation of Laboratory Animal Care international guidelines and approved by the National Cancer Institute Animal Care and Use Committee. Generation of Gm15441 -null mice SAGE Laboratories (Cambridge, UK) provided design and construction services for the CRISPR/Cas gene targeting technologies used to create a Gm15441 -null ( Gm15441 LSL ) mouse line. 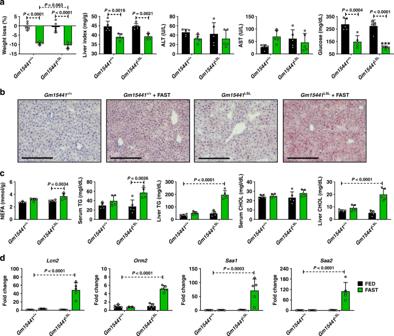Fig. 6: Loss ofGm15441potentiates inflammasome activation during physiological response to acute fasting. aPhysiological endpoints fromGm15441+/+andGm15441LSLmice after 24 h fasting. Weight loss and liver indices (mg liver/g body mass; a measure of hepatomegaly), as well as blood ALT, AST, and glucose levels, in response to fasting.bRepresentative ORO staining of liver tissues after a 24 h fed or fast inGm15441+/+andGm15441LSLmice (n= 5, 3 images/mouse). Scale bars represents 100 nm (×200).cNon-esterified fatty acid (NEFA) from serum, triglycerides (TG) and cholesterol (CHOL) levels from serum and liver tissues after a 24 h fast.dAnalysis ofApoa4,Bhmt,Lcn2,Orm2,Saa1, andSaa2mRNAs in livers ofGm15441+/+andGm15441LSLmice after 24 h fasting. Each data bar represents the mean ± SD forn= 5 liver samples; green bars, 24 h fasting. Adjustedpvalues, provided in the panels, as determined by ANOVA with Tukey’s multiple comparison correction, two-sided for comparisons between fast-stimulated and unstimulated livers of the same genotype, or as shown (dashed horizontal lines). The targeting strategy results in the insertion of a floxed cassette containing a transcriptional stop repeat within the first intron of Gm15441 (NR_040409.1) (Supplementary Table 6 ). Presence of the cassette prevents Gm15441 expression. Crossing with a Cre mouse line removes the stop cassette and allows Gm15441 expression to proceed. Microinjection-ready sgRNA, Cas9 mRNA, and a plasmid donor with a floxed stop cassette were purchased from SAGE Laboratories. The sgRNA, Cas9 mRNA, and plasmid donor were then injected into C57BL/6J mouse embryos by the Transgenic Mouse Model Laboratory at the National Cancer Institute (Fredrick, MD) using the manufacturer’s recommended protocol. 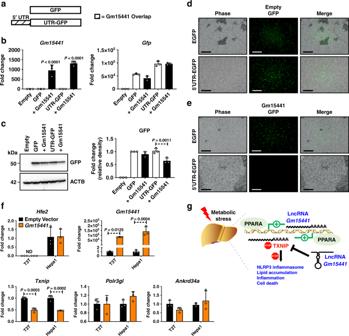Fig. 7:Gm15441regulates TXNIP translation in part through IRES sequences found within the 5′UTR of TXNIP. aSchematic representation of GFP construct inserts with or without the TXNIP 5′UTR sequence.bAnalysis ofGm15441RNA andGfpmRNA in Hepa-1 cells.cWestern blot analysis of GFP protein and relative density of GFP signal from Hepa-1 cells (right).dFluorescence of GFP in Hepa-1 cells transfected with GFP with empty orGm15441plasmid DNA for 48 h (n= 3). Scale bars represent 20 nm (100x).eFluorescence of GFP in Hepa-1 cells transfected with 5′ UTR sequence containing GFP with empty orGm15441plasmid DNA for 48 h (n= 3). Scale bars represent 20 nm (100x).fAnalysis ofHfe2,Pol3gl, andAnkrd34amRNAs from Hepa-1 and NIHT3T cells transfected with empty plasmid orGm15441expression vector for 24 h. Each data point represents mean ± SD forn= 3 replicates. Adjustedpvalues, provided in the panels, as determined by ANOVA with Tukey’s multiple comparison correction, one-sided for comparisons in the absence of Gm15441 (b,c) or to empty vector (f).gModel for role of Gm15441 in suppressing TXNIP-mediated inflammasome activation. Founder animals were genotyped using primer sets in Supplementary Table 7 , and all modifications were confirmed by targeted sequencing. Homozygous mice were then backcrossed ten times into the C57BL6 background to breed out any off-target effects. Mouse genotyping Genomic DNA was extracted from mouse tail snips using the Sigma REDExtract-N-Amp Kit. Genotyping was performed following the manufacturer’s protocol with the following modifications. Twenty five µl of E buffer and 7 ul of TPS buffer were added to each snip and the samples stored room temperature for 10 min. Samples were heated at 95 °C for 5 min then 25 µl of N buffer was added. Polymerase chain reactions for genotyping Gm15441 mice used the following primers: forward: 5′-TGCGAGGCACGATATGGCGA-3′, reverse: 5′-AGCGCACCTGTCACTTTCCTGC-3′. Bands of 1200 bp or 1700 bp were detected in wild-type and Gm15441 LSL mice, respectively. Preparation of adeno-associated virus (AAV) expressing short hairpin (sh) RNA targeting TXNIP For the TXNIP knockdown studies, AAV gene delivery vectors were constructed by cloning TXNIP shRNA sequences into an AAV-shRNA plasmid (Addgene #85741, Watertown, MA). The AAV-shRNA expression plasmid was digested with XbaI and BamHI and a shRNA sequence (5′-GGACTACTTGCGCTATGAAGA-3′) targeting the first exon of TXNIP was inserted. AAV2/8 virus was generated by transfecting HEK293T cells with the pAAV2 insert containing either shRNA control or shRNA-Txnip under the control of the mouse U6 promoter, and flanked by serotype-2 inverted terminal repeats, pXR1 containing rep and cap genes of AAV serotype-8, and pHelper encoding the adenovirus helper functions (Addgene, Watertown, MA). Cell lysates were subjected to three rounds of freeze/thaw and then treated with 1 ul of benzonase (Sigma St. Louis, MO) per 5 ml of lysate for 30 min at 37 °C and clarified by centrifugation. Virus was purified by iodixanol gradient ultracentrifugation and titered by qRT-PCR. Mice 11-12 weeks old were given AAV-shRNA- Txnip or AAV-shRNA-Ctrl at a dose of 1 × 10 12 genome copies/mouse by tail vein injection. Six weeks later, the mice were given a second AAV injection and allowed another two weeks to recover. Mice were then provided with control or WY-14643-containing diets and killed 24 h later. RNA isolation, library construction, and RNA sequencing RNeasy Plus Mini Kits (Qiagen, Valencia, CA, USA) were used to extract total RNA from livers from four different treatment and control groups, namely wild-type and Ppara −/− mice treated with control or WY-14643-containing diets. Mice were fed either control diet or fed a matching diet containing 0.1% WY-14643 for 48 h. All mice were killed between 1 and 3 PM. RNAs were extracted from n = 9 to 15 independent livers per group and RNA quality assessed using a TapeStation 4200 (Agilent, Santa Clara, CA, USA). High quality RNA samples (RIN > 9.0) were pooled, as described below, and used to construct stranded RNA-seq libraries from polyA-selected total liver RNA using an Illumina stranded TruSeq mRNA Prep Kit (Illumina, San Diego, CA, USA). Three pooled RNA samples were prepared for each of the four treatment groups with each pool comprised of n = 3-5 individual liver samples. The libraries were subjected to paired-end sequencing using an Illumina HiSeq 2500 instrument (Illumina) at the NCI-CCR sequencing facility (Frederic, USA) at a depth of 30-42 million read pairs for each of the 12 RNA-seq libraries. For RNA-seq analysis of Gm15441 LSL mice, total liver RNA was isolated from wild-type mice and Gm15441 LSL mice fed either control diet or a diet containing 0.1% WY-14643 for 24 h and killed between 1 and 3 PM. RNAs were extracted from n = 9 independent livers per experimental group, analyzed for RNA quality (RIN > 9.0), and used to prepare sequencing libraries. Three pooled RNA samples were prepared for each of the 4 treatment groups, with each pool comprised of n = 3 individual liver RNA samples. Libraries were subjected to 150 cycle paired-end Illumina sequencing at a depth of 13–21 million read pairs for each of the 12 RNA-seq libraries. Analysis of sequencing results Data were analyzed using a custom RNA-seq analysis pipeline [18] , [82] . Briefly, sequence reads were mapped to the mouse genome (release mm9) using TopHat2 (v2.1.1) [83] . Genomic regions that contain exonic sequence in at least one isoform of a gene (exon collapsed regions [82] ;) were defined for each RefSeq gene and for each lncRNA gene. HTSeq (0.6.1p1) was then used to obtain read counts for exon collapsed regions of RefSeq genes, and featureCounts (1.4.6-p5) was used to obtain read counts for exon collapsed regions of lncRNA genes. A set of 24,197 annotated mouse RefSeq genes (which includes some RefSeq lncRNAs) and a set of 15,558 liver-expressed lncRNA genes [17] , [18] was considered for differential expression analysis. These lncRNAs include intergenic lncRNAs, as well as lncRNAs that are antisense or intragenic with respect to RefSeq genes, and were discovered using a computational pipeline for lncRNA discovery described elsewhere [16] based on 186 mouse liver RNA-seq datasets representing 30 different biological conditions. RefSeq and lncRNA genes that showed significant differential expression following exposure to WY-14643 were identified by EdgeR as outlined elsewhere [16] . Genes dysregulated with an expression fold-change (i.e., either upregulation or downregulation) >2 at a false discovery rate (FDR), i.e., an adjusted P -value < 0.05 were considered significant and are shown in Supplementary Table 1 and Supplementary Table 5 . Raw and processed RNA-seq data are available at GEO ( https://www.ncbi.nlm.nih.gov/gds ) accession numbers GSE132385 and GSE132386. Cell culture and transfection Primary hepatocytes were isolated from C57BL6N mice as previously reported [84] and seeded on collagen-coated 12-well plates (Becton Dickinson and Company, Franklin Lakes, NJ) at a density of 2 × 10 5 cells in Williams’ Medium E (Thermo-Fisher Scientific, Waltham, MA) supplemented with 5% FBS and penicillin/streptomycin/amphotericin B solution (Gemini Bio-products, West Sacramento, CA). Hepa-1 mouse hepatoma cells and NIHT3T mouse embryonic fibroblast cells (ATCC, Manassas, VA) were maintained at 37 °C in a humidified atmosphere of 5% CO 2 in Dulbecco’s Modified Eagle Medium (DMEM) containing 10% Fetal Bovine Serum (FBS) and 1% of penicillin/streptomycin mixture (Invitrogen, Waltham, MA). pCMV-EGFP plasmid was purchased from Addgene (Addgene #11153, Watertown, MA). pCMV-Txnip plasmid was purchased from Origene (Origene #PS10001). Spliced Gm15441 transcript insert was cloned into pCMV-EGFP to generate pCMV-Gm15441. One day after seeding, Hepa-1 and NIHT3T cells were transfected with recombinant pCMV-Gm15441 and pCMV-Txnip for 48 h. The cells were then harvested and analyzed by qRT-PCR and western blotting. For 5′UTR transfection experiments, the 5′UTR sequence from Txnip was inserted into pCMV-EGFP plasmid followed by transfection in Hepa-1 cells for 48 h. Non-5′UTR inserted pCMV-EGFP was used as a negative control. The cells were subjected to microscopic analysis or harvested and subjected to qRT-PCR and western blotting. Histological staining Fresh liver tissue was immediately fixed in 10% phosphate-buffered formalin for 24 h and then processed in paraffin blocks. Four-micrometer sections were used for H&E staining. For Oil Red O (ORO) staining, fresh liver tissue was placed into a cryomold and filled with OCT Compound (Tissue-Tek), then transferred to a beaker of isopentane prechilled in liquid nitrogen. Sections were processed by HistoServ, Inc. (Germantown, MD). Slide imaging was performed using a Keyence BZ-X700 series all-in-one microscope with both ×20 and ×40 objectives, ×200 and ×400 magnification, respectively. Serum biochemistry Blood was collected from mice and transferred to BD Microtainer Serum Separator Tubes (Becton Dickinson, Franklin Lakes, NJ). Serum was flash frozen in liquid nitrogen and stored at -80C. Serum chemistry analysis for total cholesterol (CHOL), non-esterified fatty acids (NEFA), and triglycerides (TG) was performed using Wako Clinical Diagnostics kits (WakoUSA, Richmond, VA). Serum alanine aminotransferase (ALT) and aspartate aminotransferase (AST) levels were measured using Catachem VETSPEC Kits as recommended by the manufacturer (Catachem, Oxford, CT). Blood glucose (GLU) levels were measured using a Contour blood glucose meter (Bayer, Mishawaka, IN). Serum SAA1 analysis was performed using Mouse Serum Amyloid A Quantikine ELISA Kit (R&D Systems, Minneapolis, MN). Metabolic assays For the glucose tolerance tests (GTT), mice were fasted overnight for 16 h. For the insulin tolerance tests (ITT), the mice were fasted for 4 h. Glucose at 2 g/kg or insulin (Eli Lilly, Washington, DC) at 0.8 U/kg in saline were injected intraperitoneally into animals and blood glucose measured from tail bleeds using a Contour Glucometer (Bayer, Mishawaka, IN). Blood glucose was measured before the injection and at intervals of 15 min for 2 h post injection using the glucometer. Western blot analysis Whole-cell extracts were prepared from mouse liver tissue or mouse primary hepatocytes using RIPA buffer supplemented with Halt Protease and Phosphatase Inhibitor Cocktail (Thermo-Fisher Scientific) and 1 mM PMSF. Protein concentrations were determined using the Pierce BCA Protein Assay Kit (Pierce, Rockford, IL). Twenty to forty μg of protein lysate was loaded per lane on a 4–12% Criterion TGX Precast Gel (Bio-Rad) then transferred to PVDF membranes using a Trans-Blot Turbo Transfer System (Bio-Rad). Membranes were blocked in 5% nonfat milk followed by an overnight incubation with primary antibodies targeting TXNIP (Novus #NBP1-54578), CASP1 (Invitrogen #14-9832-82), or IL1B (Cell Signaling #12242) at 4 °C. Primary antibodies were diluted at 1:500 before use. Following primary antibody incubation, the blots were washed and incubated with HRP-conjugated secondary antibodies for one hour (Cell Signaling #7074S, #7076S). Secondary antibodies were diluted at 1:5000 before use. The blots were then stripped using Restore Western Blot Stripping Buffer (Thermo-Fisher Scientific) and re-probed with alternate antibodies. An antibody against ACTB (Cell Signaling #8457L) was used as a loading control. Blot imaging was performed on a ChemiDoc MP System (Bio-Rad) after exposing the blot to Clarity Western ECL Blotting Substrate (Bio-Rad). Protein expression was quantitatively analyzed using band density and ImageJ software (NIH, Bethesda MD) [85] . Quantitative reverse transcription PCR assays Total RNA was isolated from fresh mouse liver, mouse primary hepatocytes, and Hepa-1 cells using TRIzol Reagent (Thermo-Fisher Scientific, Waltham, MA, USA) and quantified using a NanoDrop Spectrophotometer (NanoDrop Products, Wilmington, DE, USA). Total RNA (2 μg) was reverse transcribed using All-in-One cDNA Synthesis SuperMix (BioTool, Houston, TX, USA). qRT-PCR analysis was performed using SYBR Green qPCR Master Mix (BioTool). Primers were designed for gene specificity and to cross exon-exon junctions using Primer-BLAST ( www.ncbi.nlm.nih.gov/tools/primer-blast/ ) and purchased from IDT DNA Technologies (Coralville, IA, USA) (Supplementary Table 7 ). qRT-PCR experiments were designed and performed according to Minimum Information for Publication of Quantitative Real-Time PCR Experiments (MIQE) guidelines [86] . Results are normalized to actin expression. Values given are fold over control or relative expression value, where appropriate, calculated using the 2ΔCt QPCR calculation method [87] . Luciferase reporter assays For luciferase assays, pSG5-PPARα (mouse) and pSG5-RXRA (mouse) were used for transcription factor expression [88] . Custom GeneBlocks (IDT DNA) were synthesized containing the predicted PPRE sites for Gm15441. GeneBlocks were digested and purified using a Qiagen PCR Purification Kit (Qiagen, Valencia, CA), and cloned into the pGL4.11 or pGL4.27 for PPRE reporter constructs (Promega, Madison, WI) using a BioRad Quick Ligation Kit (BioRad, Hercules, CA, USA). Prior to performing assays, all constructs were confirmed by Sanger sequencing at the NCI Center for Cancer Research Genomics Core. The phRL-TK renilla luciferase construct was used as a control to normalize for transfection efficiency. Primary hepatocytes were seeded into 12-well plates (4 × 10 4 cells/well). PPRE reporter constructs were co-transfected into hepatocytes with PPARα and RXR expression vectors. PPRE-luc plasmid containing an Acox1 PPRE site repeat was used as a positive control [89] . Empty pGL4.11 or pGL4.27 plasmids were used as negative controls. Plasmids were transfected using Lipofectamine 3000 Reagent (Thermo-Fisher Scientific). Luciferase activities were measured and plotted relative to lysate protein concentrations using the Promega Dual Luciferase Reporter (Promega) assays according to the manufacturer’s protocol. Measurements were taken on a Veritas microplate luminometer (Turner Biosystems, Sunnyvale, CA, USA). Chromatin immunoprecipitation Chromatin was prepared from hepatocytes for ChIP assays as previously described [90] . Cells were fixed with 4% paraformaldehyde for 15 min, then glycine was added to a final concentration of 0.125 M and incubated for 10 min before harvesting. Chromatin was sonicated using a Bioruptor Pico (Diagenode, Denville, NJ, USA). Chromatin preparations were subjected to ChIP using a ChIP-IT High Sensitivity Kit and Protein G Agarose Prepacked Columns (Active Motif, Carlsbad, CA, USA) using either PPARα (Abcam Ab24509) antibody, normal rabbit IgG (Cell Signaling Technologies #2729S), or Histone H3 (Cell Signaling Technologies #4620) antibody. Rabbit IgG and Histone H3 were used as negative and positive controls, respectively. DNA was purified and concentrated using MinElute Reaction Cleanup columns (Qiagen). qRT-PCR and conventional PCR were performed using 2 μl of ChIP DNA samples from the 50 μl of purified samples using gene-specific primers (Supplementary Table 7 ). Cycle threshold (Ct) values of ChIP and input samples were calculated and presented as fold change. RNA fluorescent in situ hybridization (FISH) For FISH staining of Gm15441, Gm15441 +/+ , and Gm15441 LSL mice were fed either a control diet or diet containing WY-14643 for 36 h. Livers were harvested, fixed in 4% of paraformaldehyde overnight then sent to the Molecular Pathology Laboratory at the National Cancer Institute for processing. RNA FISH experiments were performed using custom RNAscope probes and reagents developed by Advanced Cell Diagnostics (Newark, CA). Proprietary FISH probes targeted a region of Gm15441 that does not overlap with Txnip to prevent signal interference (Supplementary Table 8 ). Slide imaging was performed using Aperio ImageScope software (Leica Biosystems, Buffalo Grove, IL, USA). Tissue total lipase activity assays Liver, skeletal muscle (soleus), and inguinal white adipose tissue (IWAT) were homogenized in ice-cold PBS buffer using a Percellys bead homogenizer and 1 mm zirconia/silica beads. Tissue total lipase activity was assayed using a fluorometric lipase activity assay kit (Abcam #ab204721) following the manufacturer’s recommendations and normalized to total protein. According to the manufacturer, assay specificity has been confirmed for LPL, hormone-sensitive lipase [also known as (a.k.a.) LIPE], hepatic TG lipase (a.k.a. LIPC), and pancreatic TG lipase (a.k.a. PNLIP). Adipose TG lipase (a.k.a. PNPLA2) activity should also be detectable, although specificity has not directly been confirmed. Protein concentrations were determined using a Pierce BCA Protein Assay Kit (Thermo-Fisher). In vitro transcription-translation assay TNT T7 Quick Coupled Transcription/Translation System was used for checking transcription and translation (Promega) according to the manufacturer’s protocol. Linear pCMV-Empty, pCMV-Gm15441 (GenScript custom gene synthesis construct containing mature, spliced Gm15441 transcript; NR_040409.1), and pCMV-Txnip (Origene; MR206196; NM_023719) plasmids were used as templates. All plasmids included the T7 promoter sequence for RNA transcription. pCMV-Txnip plasmid (0.5 µg) was added to reticulocyte lysate in combination with increasing amounts (0.1, 0.3, and 0.5 µg) of pCMV-Empty or pCMV-Gm15441 plasmid. Western blots were then performed on lysates using anti-TXNIP antibody as described above. Blot imaging was performed on a ChemiDoc MP System (Bio-Rad) after exposing the blot to Clarity Western ECL Blotting Substrate (Bio-Rad). 5′ Rapid amplification of cDNA ends (5′ RACE) ExtractSTART Eukaryotic mRNA 5′-& 3′-RACE kit was used for cDNA library preparation according to the manufacturer’s protocol (Epicentre Biotechnologies, Illumina). 2 µg of total RNA from livers of mice treated with WY-14643 for 24 h was used for template. All steps followed the manufacturer’s protocol. PCR products were analyzed by Sanger Sequencing (2-ABI 3500xL and 1-3730xL DNA sequencers, Illumina) after cleanup using a PCR purification kit (Qiagen). The sequencing primers are listed in Supplementary Table 6 . Data and statistical analyses PPARα ChIP-seq data was downloaded from NCBI Gene Expression Omnibus (GSE61817). ChIP-seq data was uploaded to the Galaxy public server at usegalaxy.org for analysis [91] . More specifically, data were converted to bigwig file format using Galaxy tools. Bigwig files were then visualized using CLC workbench (Qiagen) and Integrated Genome Browser (version 9.0.0) [92] . All results are expressed as means ± SD. Significance was determined by t-test or one-way ANOVA with Bonferroni correction using Prism 7.0 software (GraphPad Software, La Jolla, CA, USA). A P value less than 0.05 was considered significant and statistical significance is indicated in the figure legends. Reporting summary Further information on research design is available in the Nature Research Reporting Summary linked to this article.